Mycobacteria modulate host epigenetic machinery by Rv1988 methylation of a non-tail arginine of histone H3 Mycobacteria are successful pathogens that modulate the host immune response through unclear mechanisms. Here we show that Rv1988, a secreted mycobacterial protein, is a functional methyltransferase that localizes to the host nucleus and interacts with chromatin. Rv1988 methylates histone H3 at H3R42 and represses the genes involved in the first line of defence against mycobacteria. H3R42me 2 , a non-tail histone modification, is present at the entry and exit point of DNA in the nucleosome and not within the regulatory sites in the N-terminal tail. Rv1988 deletion in Mycobacterium tuberculosis reduces bacterial survival in the host, and experimental expression of M. tuberculosis Rv1988 in non-pathogenic Mycobacterium smegmatis negatively affects the health of infected mice. Thus, Rv1988 is an important mycobacterial virulence factor, which uses a non-canonical epigenetic mechanism to control host cell transcription. The dynamic nature of chromatin organization allows for reversible changes in eukaryotic gene expression. The permissiveness of chromatin organization stems from epigenetic modifications of the DNA itself or of the histone proteins [1] , [2] . Each of the core histones can be modified at several amino acids and for each amino acid more than one type of post-translation modification is possible [3] , [4] . For example, histone H3 is known to be modified at >25 amino acids, and several lysines in histone H3 are known to be acetylated or methylated [5] , [6] , [7] . This variety of histone modifications and their correlation with gene activity forms the basis of the histone code [8] . The complexity of the histone code and its effect on gene expression is amplified by the large numbers of effector enzymes that modify specific amino acids of the histone proteins and the chromatin proteins that have specificity for particular histone modifications [9] . With this assortment of modifications and with each modification having the potential to affect gene expression by a unique mechanism, gene expression can no longer be considered as being in an ‘off’ or ‘on’ state. A small pool of data suggests that the epigenetic circuits within a mammalian cell also respond to bacterial infections [10] , [11] . There are reports that show host cell signalling mediates changes in the epigenetic modifications at specific gene loci in response to bacterial infection [12] , [13] . Other reports have provided proof of epigenetic modification by a bacterial protein. Legionella protein RomA methylates the host Histone H3 at Lysine 14 (ref. 14 ) and NuE, a protein from Chlamydia trachomatis , methylates both H3 and H4 (ref. 15 ). We previously identified the mycobacterial protein Rv2966c as a cytosine DNA methyltransferase that methylates cytosine predominantly in non-CpG host cell DNA [16] . Virulent species of mycobacteria interact and modulate their host cell machinery at various subcellular levels and by different mechanisms. Although several reports have documented changes in the expression of host genes [17] , our literature survey could not identify a study that had explored the possibility of a mycobacterial factor influencing host gene expression through a direct interaction with the host histone proteins. The aim of this study is to identify a mycobacterial protein(s) that interacts with a histone protein, modifies specific amino acids in it and influences the expression of a gene subset in the host upon infection. We show that the protein Rv1988, expressed only by virulent mycobacterial species, interacts with histone H3, dimethylates arginine at H3R42 and represses expression of genes that are important for immune responses against mycobacterial infection. Deletion of Rv1988 from the M. tuberculosis H37Rv strain reduces bacterial survival during infection, whereas expression of Rv1988 in non-virulent M. smegmatis provides a survival advantage during infection of peritoneal macrophages. Rv1988 not only provides a survival advantage to M. smegmatis, but also negatively affects the health of infected mice. Mycobacterial protein Rv1988 interacts with histone H3 To identify mycobacterial proteins that could interact with histone H3, recombinant 6X His-histone H3 purified from E.coli was incubated with Mycobacterium bovis BCG lysate. The mycobacterial proteins interacting with histone H3 were affinity purified using Ni-NTA beads and electrophoresed on an SDS–polyacrylamide gel electrophoresis ( Supplementary Fig. 1 ). Protein bands were cut out from the gel and identified by mass spectrometry (MS). One of the mycobacterial proteins identified in this analysis was Rv1988. Listed as a probable methyltransferase in the Tuberculist database [18] , Rv1988 is present in the pathogenic mycobacteria, M. tuberculosis and M. bovis but absent in the non-pathogenic M. smegmatis . To validate the interaction of Rv1988 with histone H3, HEK293 cells were transfected with a pcDNA3.1 construct containing the SFB (S-protein, FLAG, streptavidin-binding peptide)-tagged Rv1988 gene. Forty-eight hours post transfection, Rv1988 and its interacting partners were affinity purified using Streptavidin beads from the protein lysate and analysed by western blotting using histone H3 antibody. Vector alone (pCDNA3.1) construct was used as a control. As can be seen from Fig. 1a , affinity purification of SFB-Rv1988 from the HEK293 protein lysate pulled down histone H3, indicating that Rv1988 can indeed bind histone H3. Western blot probed with FLAG antibody (FLAG peptide is part of the SFB tag) was used to control pull-down efficiency ( Fig. 1a , lower panel). Interaction of Rv1988 with histone H3 was further confirmed by immunoprecipitation (IP) of histone H3 from the protein lysate of HEK293 cells transfected with SFB-Rv1988, followed by western blotting and probing with FLAG antibody. As a control, IP was also performed with IgG. FLAG-tagged SFB-Rv1988 was co-immunoprecipitated with H3 but not with IgG ( Fig. 1b ). IP efficiency was checked by probing the blots with antibody to histone H3 ( Fig. 1b , lower panel). 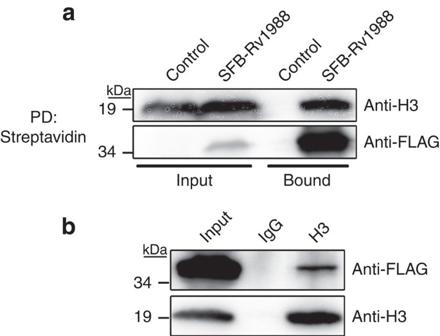Figure 1: Rv1988 interacts with histone H3. (a) Lysate of HEK293 cells, transfected with SFB-Rv1988 or pcDNA3.1 (control) constructs and pulled down with streptavidin beads was probed with antibodies as indicated. In all, 5% of the whole-cell lysate was used as Input. Streptavidin pulls down SFB-Rv1988. PD: pull down. (b) Immunoprecipitation was performed with H3 antibody on SFB-Rv1988-transfected HEK293 cells and probed with antibodies as indicated. IP was also done with IgG as a control. In all, 10% of the whole-cell lysate was used as Input. Anti-FLAG antibody detected SFB-Rv1988. Figure 1: Rv1988 interacts with histone H3. ( a ) Lysate of HEK293 cells, transfected with SFB-Rv1988 or pcDNA3.1 (control) constructs and pulled down with streptavidin beads was probed with antibodies as indicated. In all, 5% of the whole-cell lysate was used as Input. Streptavidin pulls down SFB-Rv1988. PD: pull down. ( b ) Immunoprecipitation was performed with H3 antibody on SFB-Rv1988-transfected HEK293 cells and probed with antibodies as indicated. IP was also done with IgG as a control. In all, 10% of the whole-cell lysate was used as Input. Anti-FLAG antibody detected SFB-Rv1988. Full size image Rv1988 is a functional histone methyltransferase Since Rv1988 was listed as a probable methyltransferase in the Tuberculist database [18] , we decided to test whether Rv1988 could methylate histone H3. In vitro methyltransferase assay was performed with recombinant MBP-Rv1988 using recombinant histone H3 (purified from E.coli ) as substrate and tritiated S-adenosyl methionine (SAM) as methyl group donor and analysed by autoradiography or scintillation counting. Tritiated methyl groups were transferred to histone H3 in presence of MBP-Rv1988 but not with MBP protein ( Fig. 2a ). Scintillation quantitation also indicated that statistically higher amount of tritiated methyl groups were transferred from tritiated SAM to histone H3 in presence of MBP-Rv1988 than MBP, indicating that Rv1988 can methylate histone H3 ( Fig. 2b ). Bioinformatic comparison with the human proteome database indicated that Rv1988 had some similarity with protein Arginine methyltransferases (PRMTs). As members of PRMT family are known to dimethylate arginine residues in histones [19] , we performed in vitro histone methyltransferase assay on recombinant histone H3 using cold SAM and after western blotting, probed with a dimethyl arginine antibody (Abcam ab413). Dimethyl arginine antibody detected histone H3 that was incubated with MBP-Rv1988 but not with MBP ( Fig. 2c ). Further confirmation was obtained by mutating the Adomet (SAM binding) domain of Rv1988 and performing the in vitro methyltransferase assay. In this assay, Rv1988 Adomet mutant was not able to methylate H3 ( Fig. 2c , right panel). To identify the residues within histone H3 that get methylated by Rv1988, histone H3 incubated with Rv1988 was analysed by tandem MS/MS, which indicated that arginine at the 42nd position of histone H3 (H3R42) was methylated ( Fig. 2d ). To ascertain this, arginine at H3R42 was changed to alanine by site-directed mutagenesis followed by in vitro histone methyltransferase assay using cold SAM, followed by western blotting and probing with dimethyl arginine antibody. As a control, we also mutated arginine at H3R2, H3R17 (known in literature to be dimethylated [19] ) and H3R83 (randomly selected) to alanine. H3R42A showed negligible levels of arginine methylation as compared with H3, H3R2, H3R17 and H3R83A suggesting that H3R42 was the primary target of Rv1988 ( Fig. 2e ). As seen for other histone arginine methyltransferases [20] , [21] , Rv1988 also seemed to have a minor secondary target because of which residual methylation was seen for the H3R42A mutant. This was reconfirmed by performing this assay with tritiated SAM and radiography ( Supplementary Fig. 2 ). To examine whether other histones were also methylated by Rv1988, histones were isolated from HEK293 cells, incubated with cold SAM and Rv1988, and probed with dimethyl arginine antibody. As a control, histones were also incubated with Rv1988 Adomet mutant in the in vitro methyltransferase assay. Arginine methylation was detected only for histone H3 ( Fig. 2f ). 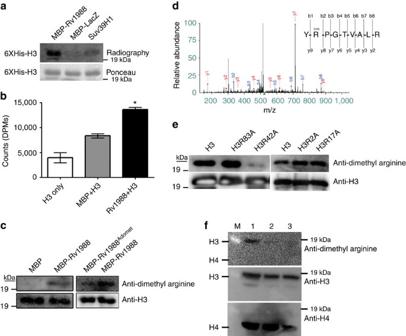Figure 2: Rv1988 is a histone methyltransferase (HMTase). (a) Autoradiogram showing histone methylation activity of MBP-Rv1988 using tritiated SAM as a methyl group donor and recombinant histone H3 as a substrate. MBP-LacZ and SUV39H1 proteins were used as negative and positive control, respectively. Ponceau staining of histone H3 was used as a loading control. (b)In vitroHMTase assay result analysed by scintillation counting. The error bars represent s.d. *Student’st-test, *P<0.05. (c) Western blot forin vitroRv1988 HMTase assay (as inabut using cold SAM) with dimethyl arginine (upper panel) and histone H3 (lower panel) antibody. SAM-binding domain was mutated in MBP-Rv1988Adomet(Methods). (d) MS/MS spectra of histone H3 peptide (amino acids 41–49) YRmePGTVALR (Arg42-methylated). In the spectra, the ‘b’ ions are labelled in blue and ‘y’ ions are labelled in red. Evidence of Arg42 methylation is provided by b2 ion at 334.187m/zand y8 ion at 883.547m/z. (e) Western blot forin vitroHMTase assay with Rv1988 and recombinant histone H3 and its mutants H3R2A, H3R17A, H3R42A and H3R83A as substrates and cold SAM as methyl group donor, probed with the indicated antibodies. (f) HMTase assay with histone proteins isolated from HEK293 cells, cold SAM and MBP-Rv1988 or MBP-Rv1988Adomet. The western blot was probed with the indicated antibodies. M: Marker (19 kDa marker band is visible); 1: histones+Rv1988; 2: histones+Rv1988Adomet; 3: histones alone. Figure 2: Rv1988 is a histone methyltransferase (HMTase). ( a ) Autoradiogram showing histone methylation activity of MBP-Rv1988 using tritiated SAM as a methyl group donor and recombinant histone H3 as a substrate. MBP-LacZ and SUV39H1 proteins were used as negative and positive control, respectively. Ponceau staining of histone H3 was used as a loading control. ( b ) In vitro HMTase assay result analysed by scintillation counting. The error bars represent s.d. *Student’s t -test, * P <0.05. ( c ) Western blot for in vitro Rv1988 HMTase assay (as in a but using cold SAM) with dimethyl arginine (upper panel) and histone H3 (lower panel) antibody. SAM-binding domain was mutated in MBP-Rv1988 Adomet (Methods). ( d ) MS/MS spectra of histone H3 peptide (amino acids 41–49) YRmePGTVALR (Arg42-methylated). In the spectra, the ‘b’ ions are labelled in blue and ‘y’ ions are labelled in red. Evidence of Arg42 methylation is provided by b2 ion at 334.187 m/z and y8 ion at 883.547 m/z . ( e ) Western blot for in vitro HMTase assay with Rv1988 and recombinant histone H3 and its mutants H3R2A, H3R17A, H3R42A and H3R83A as substrates and cold SAM as methyl group donor, probed with the indicated antibodies. ( f ) HMTase assay with histone proteins isolated from HEK293 cells, cold SAM and MBP-Rv1988 or MBP-Rv1988 Adomet . The western blot was probed with the indicated antibodies. M: Marker (19 kDa marker band is visible); 1: histones+Rv1988; 2: histones+Rv1988 Adomet ; 3: histones alone. Full size image Rv1988 is a secretory protein For Rv1988 to function as a histone methyltransferase in the host cell upon infection, the mycobacterial cell would need to secrete it. We first tested Rv1988 secretion in vitro into the culture filtrate both for M. bovis BCG and Rv1988-transformed M. smegmatis (does not have Rv1988 homologue) and grown in Sauton’s minimal media. Rv1988 (Mb2010 in M. bovis BCG) was detected predominantly in the culture filtrate of both M. bovis BCG and Rv1988-transformed M. smegmatis ( Fig. 3a,b , upper panel). GroEL1 was used as negative control for mycobacterial cell lysis ( Fig. 3a,b , lower panel). The identity of Rv1988 in culture filtrate of Rv1988-6XHis-transformed M. smegmatis was confirmed by MS of Ni-NTA affinity-purified protein present in the culture filtrate ( Supplementary Fig. 3 ). 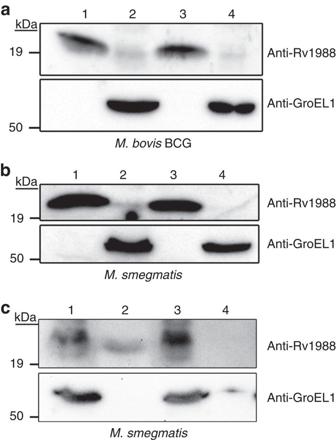Figure 3: Rv1988 is secreted by mycobacteria. Rv1988 secretion inM. bovisBCG (a) and Rv1988-transformedM. smegmatis(b). Western blot showing cell lysate and culture filtrate ofM. bovisBCG and Rv1988::M. smegmatiswas probed with Rv1988 and GroEL1 antibodies. Mb2010, Rv1988 homologue inM. bovisBCG (a) or Rv1988 (b) was detected by Rv1988 antibody (upper panel) in culture filtrate (lanes 1, 3) and cell lysate (lanes 2, 4) of two independent cultures. (c) Mutation in the Tat-signal sequence abolishes the secretory potential of Rv1988. Culture filtrate and cell lysate for Rv1988-6XHis and Rv1988R8A/R9A-6XHis-transformedM. smegmatiswas probed for the presence of Rv1988. 1: cell lysate and 2: culture filtrate for Rv1988-6XHis::M. smegmatis; 3: cell lysate and 4: culture filtrate for Rv1988R8A/R9A-6XHis::M. smegmatis. GroEL1 (a non-secretory protein) antibody was used to examine cell lysis (lower panel). Figure 3: Rv1988 is secreted by mycobacteria. Rv1988 secretion in M. bovis BCG ( a ) and Rv1988-transformed M. smegmatis ( b ). Western blot showing cell lysate and culture filtrate of M. bovis BCG and Rv1988:: M. smegmatis was probed with Rv1988 and GroEL1 antibodies. Mb2010, Rv1988 homologue in M. bovis BCG ( a ) or Rv1988 ( b ) was detected by Rv1988 antibody (upper panel) in culture filtrate (lanes 1, 3) and cell lysate (lanes 2, 4) of two independent cultures. ( c ) Mutation in the Tat-signal sequence abolishes the secretory potential of Rv1988. Culture filtrate and cell lysate for Rv1988-6XHis and Rv1988 R8A/R9A -6XHis-transformed M. smegmatis was probed for the presence of Rv1988. 1: cell lysate and 2: culture filtrate for Rv1988-6XHis:: M. smegmatis ; 3: cell lysate and 4: culture filtrate for Rv1988 R8A/R9A -6XHis:: M. smegmatis . GroEL1 (a non-secretory protein) antibody was used to examine cell lysis (lower panel). Full size image For their secretion, bacterial proteins are usually dependent upon the Sec or Tat secretion pathways [22] . Bioinformatic analysis of the Rv1988 protein sequence indicated the presence of Tat-signal sequence (Z-R-R-x-Φ-Φ) within its N-terminus ( Supplementary Fig. 4 ). To confirm the secretory nature of Rv1988 we mutated the twin arginine motif at positions R8 and R9 to a twin alanine motif. M. smegmatis transformed with Rv1988-6XHis or Rv1988 R8A/R9A -6XHis was grown in Sauton’s minimal media and the culture filtrate was tested for the presence of Rv1988. Only Rv1988-6XHis protein was detected in culture filtrate (lane 3, Fig. 3c ). Rv1988 R8A/R9A -6XHis was absent from the culture filtrate (lane 4, Fig. 3c ) confirming the secretory nature of Rv1988. Transformation with Rv1988 or Rv1988 R8A/R9A did not affect the in vitro growth of M. smegmatis in culture. Rv1988 localizes to the chromatin upon infection To confirm the secretion of Rv1988 from the mycobacterial cell into the host cell upon infection, mouse peritoneal macrophages were infected with GFP:: M. smegmatis or Rv1988-GFP:: M. smegmatis strains and the localization of GFP was examined by confocal microscopy. As shown in Fig. 4a , the GFP fluorescence was limited to within the boundary of the mycobacterial cell as visible in the bright-field view (marked by a red line in the inset panels) for GFP:: M. smegmatis -infected peritoneal macrophages. However, the GFP fluorescence was more diffused and spread throughout the cell in Rv1988-GFP:: M. smegmatis -infected peritoneal macrophages ( Fig. 4a ). The same was true for Rv1988-GFP:: M. smegmatis -infected PMA-treated THP1 cells (THP macrophages, Supplementary Fig. 5 ). 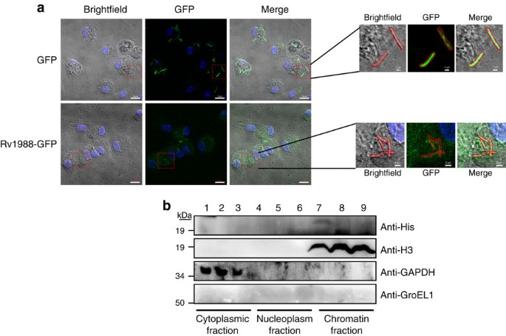Figure 4: Rv1988 localizes to the host chromatin upon infection. (a) Mouse peritoneal macrophages infected either with GFP or Rv1988-GFP expressingM. smegmatisanalysed 48 h after infection by confocal microscopy. Scale bar,∼10 μm. Inset shows a ‘zoomed in’ view of the region marked by red box. Scale bar,∼1 and 2 μm (upper and lower panel, respectively). Some of the bacilli are outlined in red. Note rod-shaped structures stained by GFP in GFP::M. smegmatis-infected peritoneal macrophages as against a diffused GFP signal in Rv1988-GFP::M. smegmatis-infected peritoneal macrophages. (b) Rv1988 localizes to the host chromatin. Subcellular fractions (as indicated below the panels) of THP1 cells infected with Rv1988-6XHis::M. smegmatis(lanes 1, 4, 7), Rv1988R8A/R9A-6XHis::M. smegmatis(lanes 2, 5, 8) or pVV16::M. smegmatis(lanes 3, 6, 9) were probed with the indicated antibodies. Histone H3 and GAPDH antibodies were used as control for chromatin and cytoplasmic fractions, respectively. GroEL1 antibody was used to show that mycobacterial cells were not lysed. Figure 4: Rv1988 localizes to the host chromatin upon infection. ( a ) Mouse peritoneal macrophages infected either with GFP or Rv1988-GFP expressing M. smegmatis analysed 48 h after infection by confocal microscopy. Scale bar, ∼ 10 μm. Inset shows a ‘zoomed in’ view of the region marked by red box. Scale bar, ∼ 1 and 2 μm (upper and lower panel, respectively). Some of the bacilli are outlined in red. Note rod-shaped structures stained by GFP in GFP:: M. smegmatis -infected peritoneal macrophages as against a diffused GFP signal in Rv1988-GFP:: M. smegmatis -infected peritoneal macrophages. ( b ) Rv1988 localizes to the host chromatin. Subcellular fractions (as indicated below the panels) of THP1 cells infected with Rv1988-6XHis:: M. smegmatis (lanes 1, 4, 7), Rv1988 R8A/ R9A-6XHis:: M. smegmatis (lanes 2, 5, 8) or pVV16:: M. smegmatis (lanes 3, 6, 9) were probed with the indicated antibodies. Histone H3 and GAPDH antibodies were used as control for chromatin and cytoplasmic fractions, respectively. GroEL1 antibody was used to show that mycobacterial cells were not lysed. Full size image Further confirmation of Rv1988 secretion into the host cell was obtained by infecting larger numbers of THP1 macrophages ( ∼ 5 × 10 7 cells) with 6X His-Rv1988-transformed M. bovis BCG. To detect Rv1988 in the host cell without lysing the mycobacterial cell wall, cell lysate was prepared in an NTEN buffer containing 0.5% NP-40 (infected mycobacterial cells are known to remain intact in this buffer [23] ) and probed for the presence of Rv1988 using 6X His antibody. Rv1988 was indeed detected in this infected THP1 cell lysate ( Supplementary Fig. 6 ). GroEL1 protein, a non-secretory mycobacterial protein, secreted was not detected in this lysate confirming that M. bovis BCG bacilli were not lysed ( Supplementary Fig. 6 , lower panel). Rv1988 localized to the nucleus when Rv1988-GFP construct was transiently transfected into HEK293 cells ( Supplementary Fig. 7 , top panel). To confirm this in an in vivo infection experiment, THP1 macrophages were infected with Rv1988-6XHis:: M. smegmatis . As a control, THP1 macrophages were also infected with pVV16:: M. smegmatis (vector control) or Rv1988 R8A/R9A -6XHis:: M. smegmatis (non-secretory mutant of Rv1988, see Fig. 3c ). Forty-eight hours after infection, subcellular fractionation of the infected THP1 macrophages [24] was performed taking care that intracellular mycobacterial cells did not lyse [23] . Rv1988-6XHis was detected only in the chromatin fraction ( Fig. 4b , lane 7, Anti-His panel). The non-secretory mutant Rv1988 R8A/R9A was not detected in any of the fractions (lanes 2, 5 and 8). H3 was used as a control for the chromatin fraction, GAPDH was used as a control for cytoplasmic fraction. Mycobacterial non-secretory protein, GroEL1, was not detected in any of the fractions confirming that M. smegmatis bacilli were not lysed. This result clearly indicated that Rv1988 is not only secreted into the host cell but has the capability to localize to the chromatin of the host nucleus. Using site-directed mutagenesis, we were also able to show that the nuclear localization of Rv1988 was dependent on three patches of basic amino acids present within the C-terminus of Rv1988 ( Supplementary Fig. 7 ). Rv1988 mediates repression through H3-arginine methylation Modification of histones especially histone H3 have been very well correlated with regulation of gene expression [3] . To examine the role of Rv1988-mediated H3R42me 2 in gene regulation, luciferase reporter gene assay was performed in HEK293 cells (Methods). If methylation of H3R42 by Rv1988 has any regulatory effect, it should change luciferase expression. Upon transfection of pG5luc with Rv1988-pBIND ( Fig. 5a ), significant decrease of luciferase activity ( ∼ 78%) was observed as compared with luciferase activity when only pG5luc alone or pG5luc+pBIND vectors were transfected ( Fig. 5b ). Furthermore, to test whether Gal4 assisted tethering of Rv1988 to the Gal4-binding sites in the luciferase promoter leads to H3R42 dimethylation, we performed ChIP analysis using dimethyl arginine antibody (R (me) 2 ) for the luciferase promoter. As a control we also examined the profile of known repressive histone H3 modifications including H3K9me 3 and H3K27me 3 . While we did not observe any enrichment or depletion of H3K9me 3 and H3K27me 3 for the luciferase promoter, significant enrichment was observed for dimethyl arginine modification in cells co-transfected with Rv1988-pBIND+pG5luc as compared with control pG5luc+pBIND co-transfection ( Fig. 5c ). The observed enrichment was indeed for arginine dimethylation in histone H3 as substantial increase in the level of histone H3 dimethylated at arginine was observed in HEK293 cells transfected with Rv1988 as compared with vector alone ( Fig. 5d ). 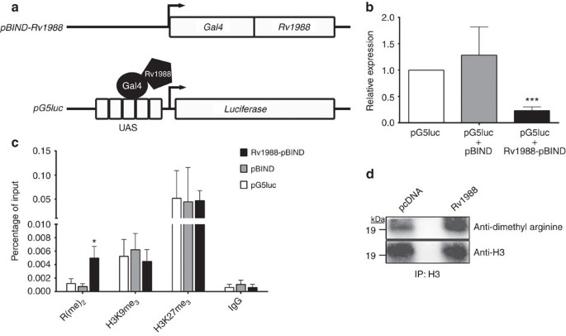Figure 5: Rv1988 mediates transcriptional repression. (a) Line diagram describing luciferase reporter gene assay strategy in HEK293 cells. The 5 UAS sites for GAL4 binding in pG5luc are shown as open rectangles. The filled shapes indicate fusion protein produced by pBIND-Rv1988 vector construct. Raised arrow indicates transcription start site. (b) Rv1988 represses transcription. Luciferase activity from pG5luc measured 48 h after co-transfection of various combinations of constructs as indicated. The values are represented as ratio w.r.t. luciferase activity of pG5luc vector alone and were normalized for transfection efficiency w.r.t. GFP expression from a co-transfected GFP construct. (c) ChIP analysis for association of various histone modifications (indicated below thex-axis) with the reporter luciferase gene promoter. Enrichment for each modification is represented as percentage input. The error bars represent s.d. Student’st-test, *P<0.05; ***P<0.0001. (d) Enrichment of H3-arginine dimethylation. ChIP performed on HEK293 cells transfected with Rv1988 or vector alone constructs using histone H3 antibody and analysed for arginine dimethylation (upper panel) and histone H3 (lower panel). Figure 5: Rv1988 mediates transcriptional repression. ( a ) Line diagram describing luciferase reporter gene assay strategy in HEK293 cells. The 5 UAS sites for GAL4 binding in pG5luc are shown as open rectangles. The filled shapes indicate fusion protein produced by pBIND-Rv1988 vector construct. Raised arrow indicates transcription start site. ( b ) Rv1988 represses transcription. Luciferase activity from pG5luc measured 48 h after co-transfection of various combinations of constructs as indicated. The values are represented as ratio w.r.t. luciferase activity of pG5luc vector alone and were normalized for transfection efficiency w.r.t. GFP expression from a co-transfected GFP construct. ( c ) ChIP analysis for association of various histone modifications (indicated below the x -axis) with the reporter luciferase gene promoter. Enrichment for each modification is represented as percentage input. The error bars represent s.d. Student’s t -test, * P <0.05; *** P <0.0001. ( d ) Enrichment of H3-arginine dimethylation. ChIP performed on HEK293 cells transfected with Rv1988 or vector alone constructs using histone H3 antibody and analysed for arginine dimethylation (upper panel) and histone H3 (lower panel). Full size image H3R42me 2 -mediated gene repression by Rv1988 during infection Two sets of genes were chosen to examine the role of Rv1988 in H3R42me 2 -mediated gene regulation during infection of macrophages by mycobacteria. First, we identified a few genomic loci in the human genome to which Rv1988 bind ( Supplementary Fig. 8 ). Of these, the sequence for region B and C ( Supplementary Table 1 ) were not repetitive in nature and present, respectively, within the intron of CDC42BPB and ENSG00000250584 , a novel lincRNA. Two immunologically important genes, TRAF3 and TNFAIP2 , were present in the same genomic locus as region B. We examined these 4 genes for their expression in GFP-Rv1988:: M. smegmatis -infected THP1 cells. Second, we observed decrease in reactive oxygen species (ROS) activity of GFP-Rv1988:: M. smegmatis -infected THP1 cells ( Supplementary Fig. 9 ). Therefore, we decided to examine the gene expression levels of a few genes known to be involved in ROS production including NOX1 , NOX4 (NADPH oxidases, involved in production of Oxygen radicals [25] ), NOXA1 (NOX-activating protein [26] ) and NOS2 (nitric oxide synthase, involved in the formation of free radicals [27] ). We first examined gene expression of the above-mentioned genes in THP1 macrophages infected with GFP:: M. smegmatis or Rv1988-GFP:: M. smegmatis by qRT-PCR. As shown in Fig. 6a , except for CDC42BPB , all other genes including the novel lincRNA, ENSG00000250584 , were repressed in Rv1988-GFP:: M. smegmatis -infected THP1 cells, confirming the repressive influence of Rv1988 on gene expression that we had earlier observed in the in vitro experiments ( Fig. 5b ). 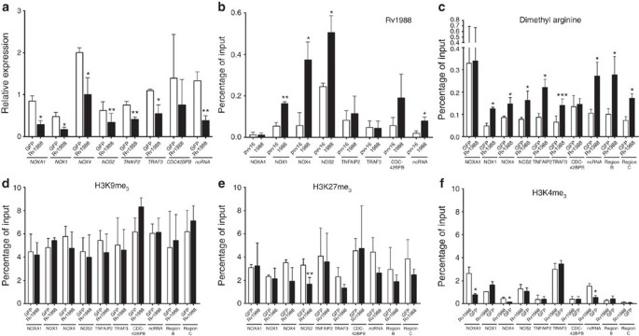Figure 6: Infection with Rv1988::M. smegmatisrepresses specific host genes. (a) Expression levels of the indicated genes measured by real-time qRT-PCR in THP1 macrophages infected withM. smegmatisexpressing Rv1988 (black bars, Rv1988) or GFP::M. smegmatis(white bars, GFP). Levels were normalized againstGAPDH. ncRNA: lincRNA ENSG00000250584. (b–f) Epigenetic modifications associated with the gene promoters. (b) Rv1988 binding; (c) dimethyl arginine; (d) H3K9me3; (e) H3K27me3; (f) H3K4me3. Region (b,c) were present within the intron ofCDC42BPBand lincRNAENSG00000250584, respectively. The error bars represent s.d. Student’st-test, *P<0.05. Figure 6: Infection with Rv1988:: M. smegmatis represses specific host genes. ( a ) Expression levels of the indicated genes measured by real-time qRT-PCR in THP1 macrophages infected with M. smegmatis expressing Rv1988 (black bars, Rv1988) or GFP:: M. smegmatis (white bars, GFP). Levels were normalized against GAPDH . ncRNA: lincRNA ENSG00000250584. ( b – f ) Epigenetic modifications associated with the gene promoters. ( b ) Rv1988 binding; ( c ) dimethyl arginine; ( d ) H3K9me 3 ; ( e ) H3K27me 3 ; ( f ) H3K4me 3 . Region ( b , c ) were present within the intron of CDC42BPB and lincRNA ENSG00000250584 , respectively. The error bars represent s.d. Student’s t -test, * P <0.05. Full size image To find whether the repression observed for these genes was associated with the binding of Rv1988 to their promoters, THP1 macrophages either infected with pVV16:: M. smegmatis or Rv1988-6XHis:: M. smegmatis were subjected to ChIP using a ChIP grade 6XHis antibody (as Rv1988 antibody was found to be good only for western blot analysis). Significant enrichment of Rv1988 was observed at the promoters of NOX1, NOX4, NOS2 and the lincRNA, ENSG00000250584 in THP1 macrophages infected with Rv1988-GFP:: M. smegmatis ( Fig. 6b ). This indicated that Rv1988 was indeed bound to the promoters of these genes. For analysing the histone H3 modifications, ChIP was also done with antibodies to dimethyl arginine, H3K4me 3 , H3K9me 3 and H3K27me 3 on THP1 macrophages infected with GFP:: M. smegmatis and Rv1988-GFP:: M. smegmatis, for the above-mentioned gene promoters, as well as for the regions B and C present within CDC42BPB and the novel lincRNA, ENSG00000250584 that we had identified to be bound to Rv1988 in our screen ( Supplementary Table 1 ). Except for NOXA1, promoters of all other genes that showed decrease in their expression in Rv1988-GFP:: M. smegmatis -infected THP1 macrophages showed significantly more association with dimethylated arginine ( Fig. 6c ). CDC42BPB expression was unaffected upon Rv1988-GFP:: M. smegmatis infection and its promoter association was also not associated with dimethyl arginine ( Fig. 6c ). No change was observed for the association of H3K9me 3 and H3K27me 3 , the known repressive chromatin marks, with the promoters of these gene upon infection with Rv1988-GFP:: M. smegmatis ( Fig. 6d,e ). In fact, NOS2 showed decrease in association with the repressive H3K27me 3 mark even though its expression level had decreased ( Fig. 6e ). Only a few of the gene promoters ( NOXA1 , NOX4 and the ENSG00000250584 lincRNA) showed decreased association with H3K4me 3 , the active chromatin-associated histone mark, in Rv1988-GFP:: M. smegmatis -infected THP1 cells ( Fig. 6f ). Both the Rv1988-bound regions B and C present within the introns of CDC42BPB and ENSG00000250584 lincRNA also showed significantly higher association with dimethyl arginine in Rv1988-GFP:: M. smegmatis -infected THP1 macrophages ( Fig. 6c ) but not with the other histone modifications tested ( Fig. 6d–f ). Control IgG ChIP is shown in Supplementary Fig. 10 . To confirm that the Rv1988 was affecting the levels of histone H3 dimethyl arginine, IP of H3 followed by western blotting with dimethyl arginine antibody was carried out on THP1 macrophages infected with Rv1988-6XHis:: M. smegmatis , pVV16:: M. smegmatis (vector control) or Rv1988 R8A/R9A -6XHis:: M. smegmatis . Significant increase in the level of H3-arginine methylation was detected only in THP1 macrophages infected with Rv1988-6xHis:: M. smegmatis ( Supplementary Fig. 11 ). To examine whether Rv1988 was also responsible for H3-arginine methylation-mediated repression of the above-mentioned genes during M. tuberculosis infection of THP1 macrophages, Rv1988 was deleted from the M. tuberculosis H37Rv strain by recombineering [28] ( Fig. 7a ). Replacement of Rv1988 region from the endogenous locus with the Hygromycin cassette was confirmed by PCR using various combinations of primers ( Fig. 7b ). The absence of Rv1988 protein from the mutant M. tuberculosis H37Rv ( ΔRv1988 ) was confirmed by western blotting using Rv1988 antibody ( Fig. 7c ). Both the strains, M. tuberculosis H37Rv and mutant M. tuberculosis H37Rv ( ΔRv1988 ), showed similar in vitro growth in culture. 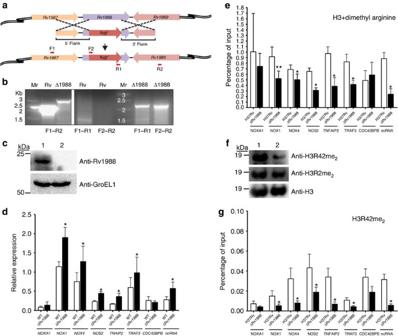Figure 7: Rv1988 is required for H3 methylation duringM. tuberculosisinfection. (a) Generation ofM. tuberculosisRv1988 gene replacement mutant. Schematic representation of the strategy used for the generation ofRv1988gene replacement mutant. (b) PCR amplifications were performed using specific primers (depicted with red arrows ina) as indicated below the agarose gel, using genomic DNA ofM. tuberculosisH37Rv andΔRv1988mutant. Left panel shows the PCR amplification with F1-R2 pair which gives a product of 2.2 kb for H37Rv and 2.9 kb forΔRv1988. Right panel shows PCR amplification with F1-R1 and F2-R2, which do not give any product with Rv genomic but yield a 2.2 kb productΔRv1988mutant. Mr: Marker, Rv:M. tuberculosisH37Rv, Δ1988:ΔRv1988mutant. (c) Absence of Rv1988 protein fromΔRv1988mutant. Western blot performed with cell lysate ofM. tuberculosisH37Rv (lane 1) andΔRv1988mutant (lane 2) was probed with Rv1988 and GroEL1 (control) antibodies. (d) Rv1988 represses specific host genes. Expression levels of the indicated genes measured by real-time qRT-PCR in THP1 macrophages infected withM. tuberculosisH37Rv (white bars, WT) orM. tuberculosisH37Rv-ΔRv1988mutant (black bars, ΔRv1988). Levels were normalized againstGAPDH. ncRNA: lincRNA ENSG00000250584. (e) Histone H3-arginine methylation by Rv1988. Double ChIP was performed, using histone H3 and dimethyl arginine antibodies (Methods), on THP1 macrophages infected withM. tuberculosisH37Rv andΔRv1988mutant. Association of histone H3, dimethylated for arginine residue, with the promoters of the indicated genes was analysed by quantitative real-time PCR. (f) Western blot to compare the H3R42me2levels between THP1 macrophages infected withM. tuberculosisH37Rv (lane 1) orΔRv1988mutant (lane 2). As a control the blot was also probed with H3R2me2and H3 antibodies. (g) Histone H3R42 dimethylation by Rv1988. ChIP was performed using histone H3R42me2antibody on THP1 macrophages infected withM. tuberculosisH37Rv andΔRv1988mutant. Association of histone H3, dimethylated at R42, with the promoters of the indicated genes was analysed by quantitative real-time PCR. The error bars represent s.d. Student’st-test, *P<0.05, **P<0.01. Figure 7: Rv1988 is required for H3 methylation during M. tuberculosis infection. ( a ) Generation of M. tuberculosis Rv1988 gene replacement mutant. Schematic representation of the strategy used for the generation of Rv1988 gene replacement mutant. ( b ) PCR amplifications were performed using specific primers (depicted with red arrows in a ) as indicated below the agarose gel, using genomic DNA of M. tuberculosis H37Rv and ΔRv1988 mutant. Left panel shows the PCR amplification with F1-R2 pair which gives a product of 2.2 kb for H37Rv and 2.9 kb for ΔRv1988 . Right panel shows PCR amplification with F1-R1 and F2-R2, which do not give any product with Rv genomic but yield a 2.2 kb product ΔRv1988 mutant. Mr: Marker, Rv: M. tuberculosis H37Rv, Δ1988: ΔRv1988 mutant. ( c ) Absence of Rv1988 protein from ΔRv1988 mutant. Western blot performed with cell lysate of M. tuberculosis H37Rv (lane 1) and ΔRv1988 mutant (lane 2) was probed with Rv1988 and GroEL1 (control) antibodies. ( d ) Rv1988 represses specific host genes. Expression levels of the indicated genes measured by real-time qRT-PCR in THP1 macrophages infected with M. tuberculosis H37Rv (white bars, WT) or M. tuberculosis H37Rv- ΔRv1988 mutant (black bars, ΔRv1988). Levels were normalized against GAPDH . ncRNA: lincRNA ENSG00000250584. ( e ) Histone H3-arginine methylation by Rv1988. Double ChIP was performed, using histone H3 and dimethyl arginine antibodies (Methods), on THP1 macrophages infected with M. tuberculosis H37Rv and ΔRv1988 mutant. Association of histone H3, dimethylated for arginine residue, with the promoters of the indicated genes was analysed by quantitative real-time PCR. ( f ) Western blot to compare the H3R42me 2 levels between THP1 macrophages infected with M. tuberculosis H37Rv (lane 1) or ΔRv1988 mutant (lane 2). As a control the blot was also probed with H3R2me 2 and H3 antibodies. ( g ) Histone H3R42 dimethylation by Rv1988. ChIP was performed using histone H3R42me 2 antibody on THP1 macrophages infected with M. tuberculosis H37Rv and ΔRv1988 mutant. Association of histone H3, dimethylated at R42, with the promoters of the indicated genes was analysed by quantitative real-time PCR. The error bars represent s.d. Student’s t -test, * P <0.05, ** P <0.01. Full size image The gene expression level of the chosen genes (as in Fig. 6a ) was quantified by qRT-PCR for THP1 macrophages infected with either M. tuberculosis H37Rv or mutant M. tuberculosis H37Rv ( ΔRv1988 ) strains. Except for NOXA1 , all genes that were repressed in THP1 macrophages infected with Rv1988-GFP:: M. smegmatis showed higher expression in mutant M. tuberculosis H37Rv ( ΔRv1988 ) strain as compared with the wild-type M. tuberculosis H37Rv strain ( Fig. 7d ). This corroborated our earlier findings ( Figs 5b and 6a ) that Rv1988 has a repressive influence on gene expression. To prove that Rv1988-mediated repression was owing to H3-arginine methylation, ChIP was performed on the chromatin from THP1 macrophages infected with either wild-type or ΔRv1988 strains of M. tuberculosis H37Rv first with H3 antibody. A second round of ChIP using the dimethyl arginine antibody was performed on the bound fraction from the H3 ChIP to obtain chromatin-associated DNA only with histone H3 having methylated arginine. As seen with Rv1988-GFP:: M. smegmatis , the promoters of all genes except NOXA1 and CDC42BPB showed significantly higher association with H3 having dimethylated arginine in THP1 macrophages infected with M. tuberculosis H37Rv as compared with infection with ΔRv1988 mutant of M. tuberculosis H37Rv ( Fig. 7e ). As a control, ChIP was also performed with IgG ( Supplementary Fig. 12 ). To further establish that during mycobacterial infection, the Rv1988-mediated methylation of arginine residues in H3 was at R42, polyclonal antibodies specific to H3R42me 2 were raised and purified ( Supplementary Fig. 13 ). Western blot analysis with this antibody showed that the level of H3R42me 2 was significantly higher in THP1 macrophages infected with M. tuberculosis H37Rv (lane 2, Fig. 7f ) as compared with ΔRv1988 mutant of M. tuberculosis H37Rv ( Fig. 7f , lane 1). In the same experiment, no significant difference was observed in the level of H3R2me 2 . To examine H3R42me 2 levels for individual genetic loci, ChIP analysis was also performed using H3R42me 2 antibody for the promoters of the selected genes (as in Fig. 7e ). Except for NOXA1 and CDC42BPB , all the gene promoters showed significant decrease in the levels of H3R42me 2 during infection with ΔRv1988 mutant of M. tuberculosis ( Fig. 7g ) mirroring our ChIP results with H3+ dimethyl arginine antibody ( Fig. 7e ). This would indicate that the repression of these genes during M. tuberculosis was being mediated through dimethylation of H3R42. Rv1988 is a mycobacterial virulence factor The ability to survive within the host macrophages is an important characteristic that differentiates the pathogenic M. tuberculosis from the non-pathogenic M. smegmatis [29] . The survivability of M. smegmatis transformed with candidate genes in macrophages has been used as an important tool to judge the importance of a gene in pathogenicity of M. tuberculosis [30] . To investigate the importance of Rv1988 during infection, we first performed infection experiments with Rv1988-transformed M. smegmatis . Mouse peritoneal macrophages in culture were infected with either Rv1988-6XHis:: M. smegmatis, Rv1988 R8A/R9A -6XHis:: M. smegmatis or pVV16:: M. smegmatis strains and the number of surviving intracellular bacilli were estimated at 0, 12, 24 and 48 h after infection. As shown in Fig. 8a , Rv1988 provided a significant survival advantage to M. smegmatis upon infection into peritoneal macrophages at all the time points for which we examined the numbers of surviving intracellular bacteria. The survival of the M. smegmatis expressing the non-secretory mutant of Rv1988, Rv1988 R8A/R9A , was significantly lower than Rv1988-6XHis:: M. smegmatis and similar to pVV16:: M. smegmatis ( Fig. 8a ). 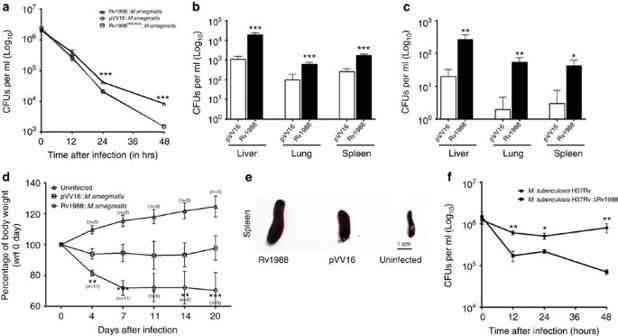Figure 8: Rv1988 is a mycobacterial virulence factor. (a) Rv1988 gives survival advantage toM. smegmatisduring infection in peritoneal macrophages. Rv1988-6XHis::M. smegmatis-, Rv1988R8A/R9A-6XHis::M. smegmatis-or pVV16::M. smegmatis-infected peritoneal macrophages cells were analysed for number of surviving internalized bacilli by CFU counting. (b,c) Survival advantage in infected mice. CFU counting was performed for various organs in BALB/c mice infected intravenously with Rv1988-6XHis::M. smegmatis(black bars) or control pVV16::M. smegmatis(white bars). A total of, 7 and 5 animals were used for each strain at the 7th (b) and 20th (c) day, respectively. (d) Rv1988-6XHis::M. smegmatisinfection negatively influences the health of the infected mice. Body weights of infected mice measured at different time points as mentioned.n=11 for both the infectedn=11 for both the infected groups till day 7.n=5 for both infected groups from day 8 to 20.n=3 for uninfected mice. Percentage of body weight for each animal was calculated with respect to their weight on the day of infection. (e) Splenomegaly in infected mice. Gross anatomy of Spleen in infected and uninfected mice as indicated. pVV16: infection with pVV16::M. smegmatis; Rv1988: infection with Rv1988-6XHis::M. smegmatis. Scale bar,∼1 cm. (f) Deletion of Rv1988 fromM. tuberculosisH37Rv reduces its survivability during infection in THP1 macrophages.M. tuberculosisH37Rv andΔRv1988mutant-infected THP1 macrophages were analysed for number of surviving internalized bacilli by CFU counting (n=3). THP1 cells were infected withM. tuberculosisH37Rv andΔRv1988strains at 1:10 MOI. The error bars represent s.d. Student’st-test, *P<0.05, **P<0.001, ***P<0.0001. Figure 8: Rv1988 is a mycobacterial virulence factor. ( a ) Rv1988 gives survival advantage to M. smegmatis during infection in peritoneal macrophages. Rv1988-6XHis:: M. smegmatis- , Rv1988 R8A/R9A -6XHis:: M. smegmatis- or pVV16:: M. smegmatis -infected peritoneal macrophages cells were analysed for number of surviving internalized bacilli by CFU counting. ( b , c ) Survival advantage in infected mice. CFU counting was performed for various organs in BALB/c mice infected intravenously with Rv1988-6XHis:: M. smegmatis (black bars) or control pVV16:: M. smegmatis (white bars). A total of, 7 and 5 animals were used for each strain at the 7th ( b ) and 20th ( c ) day, respectively. ( d ) Rv1988-6XHis:: M. smegmatis infection negatively influences the health of the infected mice. Body weights of infected mice measured at different time points as mentioned. n =11 for both the infected n =11 for both the infected groups till day 7. n =5 for both infected groups from day 8 to 20. n =3 for uninfected mice. Percentage of body weight for each animal was calculated with respect to their weight on the day of infection. ( e ) Splenomegaly in infected mice. Gross anatomy of Spleen in infected and uninfected mice as indicated. pVV16: infection with pVV16:: M. smegmatis ; Rv1988: infection with Rv1988-6XHis:: M. smegmatis . Scale bar, ∼ 1 cm. ( f ) Deletion of Rv1988 from M. tuberculosis H37Rv reduces its survivability during infection in THP1 macrophages. M. tuberculosis H37Rv and ΔRv1988 mutant-infected THP1 macrophages were analysed for number of surviving internalized bacilli by CFU counting ( n =3). THP1 cells were infected with M. tuberculosis H37Rv and ΔRv1988 strains at 1:10 MOI. The error bars represent s.d. Student’s t -test, * P <0.05, ** P <0.001, *** P <0.0001. Full size image To test whether this was also true during animal infection experiments, BALB/c mice were injected intravenously with Rv1988-6XHis:: M. smegmatis or pVV16:: M. smegmatis (control) and the bacterial load was analysed in liver, lung and spleen of the infected mice. Seven days after infection the bacterial load was found to be significantly more ( P <0.0001) for M. smegmatis that was expressing Rv1988 for all the three tissues analysed ( Fig. 8b ). The bacterial load was maximum for liver followed by spleen and was least in the lungs. This was even true 20 days after infection ( Fig. 8c ) though the total bacterial load had decreased in each tissue. While performing the animal infection experiment we noticed that there was significant body weight loss amongst mice infected with Rv1988-6XHis:: M. smegmatis . To test the significance of this observation we monitored the body weights of uninfected and Rv1988-6XHis:: M. smegmatis - and pVV16:: M. smegmatis -infected mice. As expected the uninfected mice showed increase in body weight over 20 days (Fig. 8d, n =5). While both Rv1988-6XHis:: M. smegmatis - and pVV16:: M. smegmatis -infected mice showed decrease in body weight initially (on day 4 after infection), decrease in body weight of Rv1988-6XHis:: M. smegmatis -infected mice was significantly more as compared with pVV16:: M. smegmatis -infected mice ( P <0.0001, n =16 for both groups). Subsequently (7th day onwards), pVV16:: M. smegmatis -infected mice showed signs of regaining body weight and by 20 days most of the animals in this group had more weight than on the day of the infection. However, the Rv1988-6XHis:: M. smegmatis -infected mice continued to show loss of body weight throughout and on day 20 post infection the mice in this group had on an average 35% lower weight than the pVV16:: M. smegmatis -infected mice ( Fig. 8d ). Gross examination of the various organs indicated considerable enlargement of spleen in mice infected with Rv1988-6XHis:: M. smegmatis ( Fig. 8e ). Rv1988 is present only in the pathogenic mycobacterial species like M. bovis and M. tuberculosis . To assess the importance of Rv1988 in pathogenicity, THP1 macrophages were infected with either M. tuberculosis H37Rv or M. tuberculosis H37Rv- ΔRv1988 ( ΔRv1988 mutant) and the numbers of surviving intracellular bacteria were calculated at 0, 12, 24 and 48 h after infection. As can be seen from the Fig. 8f , deletion of Rv1988 significantly reduced the number of surviving intracellular mycobacteria as early as 12 h post infection. This indicated that Rv1988 was indeed one of the virulence factor for M. tuberculosis . The outcome of an infection by a pathogenic intracellular bacteria would depend on the quantum of response that the host cell mounts against the bacteria on one hand, and the capability of the pathogen to modulate the host cellular machinery on the other. Several studies have shown examples of how the pathogenic mycobacteria uses its repertoire of proteins to modulate the host cell. Most of these proteins work at the level of cell surface and a few have been shown to interact with the host cell machinery in the cytoplasm [31] , [32] . We show here that mycobacteria upon infection secretes the protein Rv1988 in to the host cell, which then localizes to the chromatin and modulates the expression of genes important for mounting immune response against infectious bacteria through histone H3 methylation. Both in vitro histone H3 methylation assay and in vivo ChIP analysis on infected host macrophages (sequential double ChIP with H3 and dimethyl arginine antibodies, as well as a ChIP with H3R42me 2 antibody) confirmed that Rv1988 dimethylates histone H3 at R42. The interaction of Rv1988 with the host epigenetic circuitry through the non-tail core histone H3-arginine methylation (H3R42) is noteworthy because H3R42 is present at the critically important entry/exit point of DNA in the nucleosome that has the potential to change nucleosomal dynamics and affect transcription [33] , [34] . The more important point to note here is the preference of Rv1988 for a non-tail core histone H3-arginine H3R42. Mammalian histone methyltransferase normally target the lysines or arginines in the N-terminal tail of H3 including H3K4, H3K9, H3K27, H3R2, H3R8, H317 or H3R26 (refs 3 , 35 ). That bacteria use proteins to methylate histones at non-canonical sites was also borne out by the study of Rolando et al [14] who showed that RomA protein of Legionella methylates histone H3 at lysine 14, a modification not shown to be methylated in mammalian cells. Recent work from our laboratory has shown that mycobacteria use Rv2966c to methylate host DNA non-canonically predominantly at non-CpG cytosines [16] . The reason as to why pathogenic mycobacteria uses this non-canonical regulatory machinery can only be answered once we fully understand the mechanism by which methylation of H3R42 regulates transcription. A recent study showed by in vitro synthetic chromatin experiments that H3R42me 2, in presence of p53 and p300, acts to positively influence transcription [34] . On the other hand, in yeast, where a lysine is present instead of arginine at 42nd position, H3K42me 2 causes gene repression [33] . Importantly, transcription repression persisted even when this lysine was replaced with arginine [33] . Both in in vitro reporter gene assay and in vivo infection experiments, we observed, repression owing to histone H3-arginine dimethylation by Rv1988. The difference in the results could be related to the use of synthetic chromatin in vitro transcription assay [34] versus the in vitro reporter gene assay and in vivo infection studies (this study). It is also possible that the difference was owing to symmetric versus asymmetric arginine dimethylation that is known to have opposite effects on transcription [36] , [37] . Structure-based characterization of methyltransferase activity of Rv1988 would be able to shed light on this difference. Decrease in ROS activity in THP1 macrophages infected by Rv1988:: M. smegmatis strain indicated that the expression of Rv1988 in the infecting M. smegmatis had triggered the attenuation of the host machinery involved in ROS production considered to be the first line of defence against infectious agents [38] . The decrease in ROS activity correlated with Rv1988-binding and H3-arginine methylation-associated decrease in the expression of NADPH oxidase ( NOX1 and NOX4 ) and nitric oxide synthase ( NOS2 ) genes. Components of the free-radical-generating machinery were not the only factors that were targeted by Rv1988. TRAF3 , the TNF receptor-associated factor, plays an important role in both B-cell and T-cell dependent immune response [39] . The histone H3-arginine methylation-dependent transcriptional repression of TRAF3 in Rv1988:: M. smegmatis- infected THP1 cells indicated that mycobacteria uses Rv1988 to target specific genes important in mounting an immune response. This was also supported by our finding that the association of these promoters with H3R42me 2 was significantly higher during infection of THP1 macrophages with M. tuberculosis H37Rv as compared with the M. tuberculosis -Δ Rv1988 strain. The mechanisms by which these genes are targeted and the reasons why these genes are targeted would be the next step in understanding how Rv1988 modulates gene expression through its interaction with the host epigenetic circuitry. NOXA1 , a protein involved in ROS production and TNF2AIP , a protein regulated by TNFα showing repression that did not correlate with H3-arginine methylation could be indicative of repression at this loci as a secondary effect of Rv1988 action. The identification of the complete subset of genes targeted by Rv1988 is an important question that needs to be addressed. However, the aim of our study was to show that a mycobacterial protein could modulate host genome by directly interacting with its chromatin, that Rv1988 is able to methylate histone H3 at a non-canonical Arginine (H3R42) and that this modification is able to repress a subset of immunologically important genes confirms our contention. Apart from gene promoters, we have also shown H3-arginine methylation at intragenic sites that were identified as Rv1988-bound sites ( Fig. 6c ). This could suggest targeting of regulatory elements in the host genome by Rv1988. Our hypothesis was strengthened by the fact that while Rv1988-bound ‘region B’ within the CDC42BPB intron showed increased association with dimethyl arginine in THP1 cells infected with Rv1988:: M. smegmatis , the expression of CDC42BPB itself was not altered. On the other hand, the association with H3 dimethyl arginine and repression was observed for TNFAIP2 and TRAF3 , genes that are present almost 300–500 kb away from region B, indicating that the region within CDC42BPB probably was a regulatory element for TRAF3 and TNFAIP2 . Moreover, the finding that the expression of lincRNA ENSG00000250584 was also altered fits well with the known regulatory role of lincRNAs [40] . Several M. tuberculosis proteins have been shown to be important for its virulence as judged by decrease in survivability of M. tuberculosis strains deleted for the specific gene or increase in survivability of the non-pathogenic mycobacterial species, M. smegmatis , expressing these genes, within the host macrophage cell [29] , [30] . Most of these proteins are located on the mycobacterial cell surface, while some have been shown to be secreted in to the host cytoplasm [31] , [32] . The secretion of Rv1988 into the host was beneficial for the mycobacterium as the survival of M. smegmatis , which is known to be cleared very quickly from the macrophage both in vitro and in animal infection studies, was significantly better when it was expressing Rv1988. The survival ability of Rv1988:: M. smegmatis in the various tissues during animal infection studies was also markedly improved and was reflected in the diminished health of the infected animals as even 20 days after infection they were not able to regain their body weight. In addition, M. tuberculosis H37Rv strain deleted for Rv1988 was found to have significantly less survival ability after infection inside the macrophages. As epigenetic modifications play a crucial role in maintaining the transcription profile of a mammalian cell, epigenetic effectors including histone modifiers are important for the well-being of a cell. Several examples are known especially from the field of cancer where changes in the epigenetic and transcriptional profile of a cell are correlated with nuclear reprogramming and aberrant cell function [41] . The reduced survivability of M. tuberculosis H37Rv- ΔRv1988 mutant, increased survival potential of Rv1988:: M. smegmatis and negative impact of Rv1988 on the health of the infected animal suggests that its action as a histone methyltransferase had affected the epigenetic landscape of the infected cells and the animal was finding it difficult to overcome this challenge leading to decreased fitness. In summary, ours is the first report of a mycobacterial protein that acts directly at the level of host chromatin, methylates histone H3 at a non-canonical arginine residue (H3R42) present within its core-structured region, represses immunologically important genes and adversely affects the health of infected mice. Methylation of a crucial arginine, placed at the entry/exit point of DNA in the nucleosome and not within the known epigenetically important N-terminal tail of histone H3 indicates use of a novel mechanism by the pathogenic mycobacterium to subdue the host cell. This perhaps also could be one of the reasons why the host cell is not able to respond effectively when infected by a pathogenic mycobacterium species. Identification of Rv1988 as an important mycobacterial virulence factor, which uses an epigenetic mechanism to control transcription through a non-canonical mechanism, augurs well for it to be a potential target for therapy against mycobacterial infections. Purification of H3-interacting proteins from M. bovis BCG To identify M. bovis BCG proteins that interact with histone H3, E. coli- purified 6X His-tagged histone H3 was allowed to bind to pre-equilibrated Ni-NTA beads in buffer containing 50 mM Tris-HCl, pH 8, 100 mM NaCl, 1% NP-40 and 10% Glycerol, followed by incubation with pre-cleared M. bovis BCG lysate for 4 h. Ni-NTA beads alone were also incubated with M. bovis BCG lysate as control. Beads were washed five times with the same buffer but containing 25 mM Imidazole. Bound proteins were resolved on a 12% SDS–polyacrylamide gel electrophoresis. The prominent bands present only in H3 incubated fraction were cut and analysed by MS. Pull-down and IP assays Rv1988 having N-terminal SFB-tag was cloned into pCDNA3.1 and transfected into HEK293 cells (a kind gift from Dr Gayatri Ramakrishna, who obtained it from the Cell Culture Stock Centre at National Centre for Cell Science (NCCS), Pune). Forty-eight hours after transfection, cells were lysed in a buffer containing 20 mM Tris-HCl, pH 8.0, 100 mM NaCl, 1 mM EDTA, 0.5% Nonidet P-40, 50 mM β-glycerophosphate, 10 mM NaF and protease inhibitors. Lysate was incubated with pre-equilibrated Streptavidin beads for 3 h, the beads were washed five times with the same buffer, loaded on a SDS–polyacrylamide gel electrophoresis after resuspending them in 6 × -SDS sample loading buffer and western blotted. The blot was probed with H3 antibody (Abcam). For reverse IP, same procedure was followed except IP was done with H3 and IgG (Invitrogen) antibodies and probed with anti-FLAG (Sigma) antibody. Site-directed mutagenesis Site-directed mutagenesis was performed to derive the following mutants: For Rv1988: i Adomet mutant—was generated by mutating Asp38 (GAC) to Gly38 (GGC) and Gly40(GGC), Gly42(GGC) and Gly44(GGG) to Ala(GCG) using PCR-based site-directed mutagenesis. ii TAT mutant—was generated by mutating Arg8(CGA) and Arg9(CGG) to Ala8(GCA) and Ala9(GCG). For histone H3: i Arginine at 2, 17, 42 and 83 to Alanine. Histone methyltransferase assay In vitro histone methyltransferase assay was performed by incubating 2 μg of recombinant Rv1988 protein with 1–2 μg of recombinant histone H3 or its mutants and 0.2 mM cold SAM (NEB) or 2 μCi 3 H-SAM (American Radiolabelled Chemicals) in buffer containing 50 mM Tris-HCl (pH 8.0), 10% glycerol, 5 mM MgCl2, 20 mM KCl and 1 mM PMSF at 30 °C overnight. The reaction mixture was resolved on a SDS–polyacrylamide gel electrophoresis, electroblotted on polyvinylidene fluoride membrane (GE Healthcare) sprayed with Enhancer Spray (Perkin Elmer) and kept for exposure for 7 days at −80 °C. For scintillation counts, reaction was stopped by adding 10% TCA and mixture was spotted on GF/C filters (Sigma) using vacuum manifold and washed thrice with 10% TCA and twice with absolute Ethanol. Filters were dried and put in vials containing scintillation fluid and counts were taken in a scintillation counter (Perkin Elmer). Mass spectrometry After the methyltransferase assay, samples were resolved on a SDS–polyacrylamide gel electrophoresis, bands were cut and send for MS (was performed either at CDFD’s in-house mass spectrometer (Bruker) or Taplin Mass spectrometric Facility, Harvard, USA) or MS/MS (Taplin Mass spectrometric Facility). Transfection and localization of GFP-tagged proteins Rv1988 cloned into pEGFP-C3 or pEGFP-C3 alone (control) were transfected in HEK293 cells using Lipofectamine 2000 (Invitrogen). Forty-eight hours after transfection, the cells were fixed with 3.7% formaldehyde (Sigma) for 10 min, permeabilized using 0.1% triton-X-100 and mounted by using DAPI containing Vectashield mounting media (Invitrogen). Cells were visualized under a confocal microscope (Zeiss). Preparation of mycobacterium culture filtrate The culture filtrate preparation for M. bovis BCG and M. smegmatis was done as described below. To obtain Rv1988-transformed M. smegmatis , electrocompetent M. smegmatis were transformed with 1 μg DNA construct of pVV16-Rv1988 as per standardized protocol [42] . Colonies obtained after 3 days were inoculated in 5 ml Modified Sauton’s media with kanamycin and hygromycin (Invitrogen). Secondary cultures were derived using 1% primary inoculum in Modified Sauton’s media. Cultures were collected at 0.8 (OD 600 ) by centrifugation at 8,000 r.p.m. for 30 min. The supernatant was passed through 0.45 μm filters to remove cell contamination remains and concentrated 100 × using 10 kDa Centricon (Millipore). Cell lysate was prepared by sonication. Glass beads were added to the lysate during the sonication for better yields. Rv1988 antibody was raised against the E. coli -purified Rv1988 protein in mice. The specificity of the antibody was confirmed by peptide competition assay ( Supplementary Fig. 14 ). Generation of M. tuberculosis Rv1988 gene replacement mutant The 5′ homology sequence (−880 to 100 bp) and the 3′ homology sequence (438 to +851 bp) of Rv1988 were amplified from the H37Rv genomic DNA with the help of specific primers and phusion DNA polymerase. The primers for the flanks were designed such that PflMI digestion would results in ends that are compitable for cloning with hyg r cassette (amplified using specific primers) and oriE+ cosλ fragments generated from pYUB1474 construct (a kind gift from Drs William Jacobs and Apoorva Bhatt [43] ). In addition to the PflMI site, we have inserted a SnaBI site in the 5′ flank forward and 3′ flank reverse primers. Amplicons of 5′ homology sequence, 3′ homology sequence and hyg r cassette were digested with PflMI and ligated with oriE+ cosλ fragment from pYUB1474 to generate AES. AES was digested with SnaBI to generate linear allelic exchange substrate for the recombineering. M. tuberculosis H37Rv was electroporated with pNit-ET (a kind gift from Dr Eric Rubin [44] ) to generate recombineering proficient H37Rv::pNit-ET strain. H37Rv::pNit-ET cultures were grown till A 600 of 0.4 and the expression of recombineering genes were induced by the addition of 0.5 μM isovaleronitrile and the cultures were allowed to grow till A 600 of 1.0. Electrocompetent cells were prepared as described previously [28] and the cells were electroporated with 100 ng of linear allelic exchange substrates and colonies were selected on 7H11 agar plates containing 100 μg ml −1 hygromycin. Few of potential mutants obtained were cultured and genomic DNA was isolated. To confirm genuine gene replacement mutant, the potential mutants were screened using specific primers ( Fig. 7a,b ). The M. tuberculosis work was performed in the P3 facility of National Institute of Immunology, Delhi, India as per approved IBSC guidelines. Infection of THP1 cells and peritoneal macrophages In all, 0.3 × 10 6 THP1 cells (obtained from ATCC) were seeded per chamber and treated for 12 h with 10 ng of PMA. After 24 h of recovery in PMA-free RPMI medium, infection was done with different strains of M. smegmatis or M. bovis BCG in antibiotic-free media at an MOI of 30:1 for 6 h. Cells were washed twice with PBS and cultured further in media containing antibiotics. Cells were fixed or assayed at different time points as indicated. Peritoneal exudates cells were collected from BALB/c mice as per the approved IEAC guidelines (PCD/CDFD/15) and seeded in 12-well culture dishes or chamber slide at a density of 0.5 × 10 6 and 0.3 × 10 6 , respectively. Infections were done as described above for THP1 cells. For infection with M. tuberculosis , H37Rv and ΔRv1988 strain were grown up to an OD of 0.8. Bacterial cells were washed twice with PBS and were finally re-suspended in 10 ml of RPMI medium. Smooth bacterial suspension was made by passaging the cells 10 times through 27 1/2 G needle syringe. The OD was re-checked and infection was done at 1:10 MOI. The infection was allowed for 4 h and was followed by addition of media containing gentamycin for 2 h to remove extracellular bacteria. Each time point for infection with both strains was represented by three wells. At each time point cells were lysed in 1 ml 0.1% triton-X-100 and three dilutions of each were plated on plain 7H11 plates. The CFUs hence obtained after incubation at 37 °C were counted. Mice All animal experimentation was in accordance with the guidelines of CPCSEA Government of India at VIMTA Labs Limited, Hyderabad. The protocol was approved by the Institutional Animal Ethics Committee (IAEC) of the Vimta Labs (IAEC protocol approval number: PCD/OS/17 dated 14 June 2014). BALB/c mice, initially procured from Indian Institute of Science, Bangalore, India and bred in-house were used in these experiments. Mouse infection Four-to-six-week-old male BALB/c mice were injected intravenously (tail vein) with different strains of M. smegmatis (using ∼ 2 × 10 7 bacteria) as per the approved IEAC guidelines (PCD/CDFD/17). Seven days or 20 days post infection, mice were killed. To examine the bacterial load in lung, liver and spleen, the organs were homogenized in 1 ml PBS. Body weight of the individual mice was also taken at different times after infection as indicated. CFU estimation For peritoneal macrophages and THP1 cells, cells were washed twice with PBS and incubated in PBS containing 0.2% triton-X-100 for 10 min for lysis. After lysis serial dilutions were made and 100 μl from each dilution was plated on 7H10 agar containing hygromycin and kanamycin. After 3 days colonies were counted, the exact CFU count was obtained by applying the dilution factor. For CFU calculation in mice infection experiments, homogenized tissues were re-suspended in 1 ml PBS, followed by serial dilution and 100 μl from each dilution was plated on 7H10 agar containing hygromycin and kanamycin. ROS assay PMA-treated THP1 cells or peritoneal macrophages were infected with different M. smegmatis strains as described earlier. For ROS estimation equal numbers of infected THP1 cells were collected at different time points washed twice with PBS and re-suspended again in 100 μl PBS. 1 μM H 2 DCFDA (Sigma) was added to the cell suspension and incubated for 40 min in dark at 37 °C. Cells were again washed and re-suspended in PBS and DCF fluorescence was taken at 488/510 nm excitation and emission, respectively, in 96-well plate [45] . Luciferase reporter gene assay Rv1988 was cloned into pBind vector (Promega) containing Gal4 domain. pG5Luc vector was used as a reporter Luciferase construct that contains UAS sites (Gal4 binding) upstream of the Luciferase reporter gene. pEGFP-C3vector was used as a control for transfection efficiency. HEK293 cells were transfected using lipofectamine 2000 (Invitrogen), with either of the following three combinations (i) Rv1988-pBind+pG5Luc+pEGFP-C3; (ii) pBIND+pG5Luc+pEGFP-C3; (iii) pG5Luc+pEGFP-C3. After 48 h of transfection whole-cell lysate was prepared and Luciferase activity was measured using Luciferase assay system as per the manufacturer’s protocol (Promega). The same lysate was also probed with GFP antibody (Sigma) to monitor the transfection efficiency. Densitometry of the blot was done and values for GFP were used to normalize the respective luciferase values. Expression analysis by real-time PCR THP1 cells were infected with various strains of M. smegmatis and collected 48 h post infection followed by RNA isolation using TRI reagent (Sigma). In all, 1 μg DNase-treated RNA was used for cDNA preparation using Superscript III (Invitrogen). Expression analysis by real-time RT-PCR using SYBER Green Master Mix (Thermo Scientific) in ABI Prism SDS 7500 system. C t were normalized with C t of GAPDH which was used as internal control. Each experiment was done in duplicates and repeated with three biological replicates. The primers used were as following: NOXA1F 5′-ACGTCCTGTGTGAAGTGGACC-3′ NOXA1R 5′-ATGGACACAGCATCATTAGGGC-3′ NOX1F 5′-AATCCTTGGGTTTTGCAGCC-3′ NOX1R 5′-GTCGTGTTTCGGGACTGGAT-3′ NOS2F 5′-AAGCAGCAGAATGAGTCCCC-3′ NOS2R 5′-CCTGGGTCCTCTGGTCAAAC-3′ TNFAIP2F 5′-TACCCTGACTTCAGCAAAGGC-3′ TNFAIP2R 5′-CACAGGAAAAGCTAACCAACCT-3′ TRAF3F 5′-ATGATCGCGCTGCAGGTTT-3′ TRAF3R 5′-TGTCTGCTTCCTCCCAGTTC-3′ CDCBPBF 5′-GACGCACACTGTCAGAGGAA-3′ CDCBPBR 5′-GCTTCTGTATGAACTTCCAGCTCT-3′ ncRNAF 5′-AGGTACCCAGCTCCTAGCAA-3′ ncRNAR 5′-CCAGAGAGCAACAGGCATCA-3′ GAPDHRTF 5′-ACCTGCCAAATATGATGAC-3′ GAPDHRTR 5′-TCATACCAGGAAATGAGCTT-3′ Chromatin IP For ChIP using various Histone H3 and histone-modification antibodies we followed Abcam X-ChIP protocol ( http://www.abcam.com/protocols/cross-linking-chromatin-immunoprecipitation-x-chip-protocol ) with slight modifications. Briefly cultured cells were cross-linked with 0.75% formaldehyde for 10 min at room temperature followed by incubation with 125 mM of Glycine for 5 min. Cells were washed with PBS and sonicated in the ChIP lysis buffer containing 50 mM HEPES-KOH pH 7.5, 140 mM NaCl, 1 mM EDTA pH 8, 1% Triton X-1000, 1% Sodium Deoxycholate, 0.1% SDS and protease inhibitors using Bioruptor (Diagenode). In all, 50 μg of protein supernatant was taken for each ChIP and diluted 10 times with RIPA buffer (50 mM Tris-HCl, pH 8, 150 mM NaCl, 2 mM EDTA, pH 8, 1% NP-40, 0.5% sodium deoxycholate, 0.1% SDS and protease inhibitors (added freshly each time)). In all, 2 μg of the respective antibodies (5 μg for dimethyl arginine) were added to the respective samples and binding was done overnight. Twenty microliters of protein A/G (Santa Cruz) or protein-A magnetic beads (Diagenode) were added for 3 h. The beads were washed 3 times with wash buffer (0.1% SDS, 1% triton-X-100, 2 mM EDTA, pH 8, 150 mM NaCl, 20 mM Tris-HCl, pH 8)and once with final wash buffer (0.1% SDS, 1% triton-X-100, 2 mM EDTA, pH 8, 500 mM NaCl, 20 mM Tris-HCl, pH 8). The chromatin was eluted by adding 120 μl of elution buffer (1% SDS and 100 mM NaHCO 3 ) and reverse cross linked by using Proteinase K at 65°C for 4 h. The DNA was extracted by phenol:chloroform and ethanol precipitation (in presence of glycogen) followed by real-time qPCR using the following primers: NOXA1chipF 5′-CATCGGGGCCTCAGTTTC-3′ NOXA1chipR 5′-GCGCCGGATAAAGCCCT-3′ NOX1chipF 5′-CACGCTTCCCTCCCTACTTC-3′ NOX1chipR 5′-AGGGTTTTACCTGTGGGGAT-3′ NOX4chipF 5′-GAGGAAGGGTGGGAGAAACG-3′ NOX4chipR 5′-CCAGGCTCCAAAATACTGGC-3′ NOS2chipF 5′-TAAAACCTGGCTCCGTGGTG-3′ NOS2chipR 5′-TTTCCAAAGGGAGTGTCCCC-3′ TNFAIP2chipF 5′-GTCCCCCGAACTCCACATAC-3′ TNFAIP2chipR 5′-GCAAGGCCTGAAATAGTCGC-3′ TRAF3chipF 5′-CCAGCCAGGACAGCGTATTT-3′ TRAF3chipR 5′-GTTAGAGGCGACTGCCTGAG-3′ CDCBPBchipF 5′-CGGACCCCGAATACTGAAG-3′ CDCBPBchipR 5′-GTAGGGAGCCGGGATGCT-3′ ncRNAchipF 5′-AATGAGCACCCTGTCCAAAT-3′ ncRNAchipR 5′-CTCCCAGAGGACAAAAGCAG-3′ RegionBchipF 5′-ACGAGGTCAGGAGTTCGAGA-3′ RegionBchipR 5′-TGAGCCATAGCGCCTGTAAT-3′ RegionCchipF 5′-AGGTACCCAGCTCCTAGCAA-3′ RegionCchipR 5′-TGCCCATGACCTTCATTCCA-3′ LUCchipF 5′-CCGAGTTTCTAGACGGAGTACTGT-3′ LUCchipR 5′-CCCACCCCCTTTTATAGCC-3′ Each experiment was done in duplicates and repeated with three biological replicates. Antibodies GroEL1 antibody was a kind gift from Dr Shekhar Mande, NCCS, Pune, India. H3 (ab1791), H3K4me 3 (ab8580), H3K9me 3 (ab8898), H3K27me 3 (ab6002), dimethyl arginine (ab413), His (ab9108) and GAPDH (ab22555) antibodies were purchased from Abcam. The Flag antibody was purchased from Sigma (F1804). H3 antibody was purchased from Millipore (07-690). The specificity of 6XHis antibody was checked by western blotting ( Supplementary Fig. 15 ). H3R42me 2 antibody was raised against the R42 peptide ‘KPHR*YRPGTVALRC’ from histone H3, where R* corresponds to arginine R42 in H3 and was dimethylated asymmetrically (Abgenex, India). The specificity of the purified antibody (see next section for purification details) was confirmed by peptide competition assay ( Supplementary Fig. 13 ). Briefly, different concentrations of recombinant histone H3 incubated with 2 μg Rv1988 in presence of cold SAM were electrophoresed on an SDS–polyacrylamide gel electrophoresis. One set was probed with H3R42me 2 antibody pre-incubated with the methylated R42 peptide and other set was probed with H3R42me 2 pre-incubated with the unmodified R42 peptide. The peptide concentration used for competition was 1:3 (1 μg of antibody with 3 μg of peptide). The antibody was used at a dilution of 1:2,500 for 3 h at room temperature in western blotting. Antibodies against dimethyl arginine (as used in Fig. 5c ), as well as histone modifications (with the exception of H3R42me 2 ) were used at 2 μg per ChIP reaction. Apart from Fig. 5c , in all other experiments, dimethyl arginine antibody was used at 5 μg per ChIP reaction. H3R42me 2 and 6XHis antibodies were used at 3 μg per ChIP reaction. For western blots, the various antibodies were used at the following dilutions: anti-FLAG—1:5,000, anti-H3—1:4,000, anti-dimethyl arginine—1:2,500, anti-Rv1988—1:2,500, anti 6XHis—1:4,000, anti GAPDH—1:5,000 and anti H3R42me 2 —1:4,000. Purification of H3R42me 2 antibody Peptides used for antibody generation: Control peptide KPHRYRPGTVALRC Modified peptide KPHR*YRPGTVALRC (R* asymmetric dimethylation) Approximately, 10–12 ml of selected serum was taken and filtered through a Whatman filter paper. Filtered serum was then diluted with PBS in 1:1 ratio. This was mixed with non-dimethylated peptide-conjugated matrix (sulfo-link) and column was incubated on a shaker for 4 h at 25°C. This step was carried out to remove all the non-dimethylated specific antibody. After the binding of antibody, column was washed with six-column volume of PBS to wash away non-bound components of the sample solution. The flow-through was saved for purification of antibody against di-methyl peptide and was mixed with di-methyl peptide-conjugated matrix (sulfo-link) and column was incubated on shaker for overnight at 4°C. After the binding of antibody, column was washed with six-column volume of PBS to wash away non-bound components of the sample solution. Protein was eluted by passing desired amount of elution buffer (0.1 M glycine, pH 2.7) through the column. Separate 1 ml fractions were collected, neutralizing each one by prior adding 100 μl of neutralization buffer (1 M Tris-HCl, pH, 8.0, 1.5 M NaCl, 1 mM EDTA, 0.5% sodium azide). Eluted fractions of interest were pooled and dialysed into a one litre PBS with one change for overnight or the downstream application. Concentration was measured and ELISA was performed on each antibody so as to verify each lot. Uncropped scans for the gels using H3R42me 2 antibody are shown in Supplementary Fig. 16 . Identification of Rv1988-bound regions from HEK293 cells HEK293 cells transfected with pCDNA-SFB-1988 or pCDNA-SFB were processed as mentioned above in the ChIP protocol. First pull-down was done with Streptavidin beads and enriched fraction was incubated with S-protein-binding beads. The enriched DNA was end-repaired using Klenow fragment (NEB), adaptor ligated with the following annealed adaptors LK102 5′-GCGGTGACCCGGGAGATCTGAATTC-3′ and LK103 5′-GAATTCAGATC-3′ (Nimblegen Systems) PCR was performed using LK102 adaptor as primer with high fidelity Phusion High fidelity DNA Polymerase (Finnzymes). The PCR reaction was resolved on 1.5% agarose gel. Observed differentially amplified band was cut and eluted. The DNA was digested with EcoRI enzyme (NEB) and ligated in EcoRI digested pbSK vector (Stratagene). After transformation individual colonies were screened and positive clones were sequenced ( Supplementary Fig. 8 ). How to cite this article: Yaseen, I. et al. Mycobacteria modulate host epigenetic machinery by Rv1988 methylation of a non-tail arginine of histone H3. Nat. Commun. 6:8922 doi: 10.1038/ncomms9922 (2015).